Acid sensing by sweet and bitter taste neurons inDrosophila melanogaster Drosophila melanogaster can taste various compounds and separate them into few basic categories such as sweet, bitter and salt taste. Here we investigate mechanisms underlying acid detection in Drosophila and report that the fly displays strong taste aversion to common carboxylic acids. We find that acid tastants act by the activation of a subset of bitter neurons and inhibition of sweet neurons. Bitter neurons begin to respond at pH 5 and show an increase in spike frequency as the extracellular pH drops, which does not rely on previously identified chemoreceptors. Notably, sweet neuron activity depends on the balance of sugar and acid tastant concentrations. This is independent of bitter neuron firing, and allows the fly to avoid acid-laced food sources even in the absence of functional bitter neurons. The two mechanisms may allow the fly to better evaluate the risk of ingesting acidic foods and modulate its feeding decisions accordingly. In animals, the taste system is important not only for detecting nutritious foods but also as a first line of defense against ingesting noxious stimuli [1] . Many animals thus have innate taste-driven avoidance behaviours to compounds that are potentially harmful, including allelochemicals, alkaloids and acids [1] . Carboxylic acids are widely found in nature and high acidity is often associated with unpalatable foods [2] . However, the mechanisms by which acid tastants are detected, including in the model insect D. melanogaster , are poorly understood. Taste sensing in both mammals and flies is organized in a few cell types that are specialized to detect various categories of tastants and convey either acceptance or rejection [1] . In the fly, neurons for sweet and bitter stimuli express members of the large, divergent gustatory receptor (Gr) family [3] , [4] . Individual Grs expressed in these neurons have been linked to detection of sugars and polyols [5] , [6] , [7] , [8] , [9] , or alkaloids and other bitter compounds [10] , [11] , [12] , [13] . Bitter-sensing neurons also express nociceptors of the transient receptor protein family, such as TrpA1 and painless, which mediate responses to reactive electrophiles [14] , [15] , [16] . Previous studies have identified additional classes of taste neurons that detect osmolarity [17] , [18] , salts [19] , carbonation [20] and pheromones [21] , [22] , [23] , [24] . However, those that detect acids have not yet been identified. Taste receptor cells that are selectively activated by acidic or sour stimuli have been found in mammals. These cells are labelled by polycystic kidney disease-like channels, PKD2L1 and PKD1L3, and are necessary for physiological and behavioural responses to acidic stimuli [25] , [26] . However, mice lacking PKD2L1 and PKD1L3 show only a partial reduction in acid sensitivity [27] , indicating the presence of other molecular acid sensors in these taste cells. A more recent study showed that responses to acidic stimuli are mediated by proton conductance, which is blocked by zinc but not by other agents that are known to block proton channels [28] . Previous studies in the blowfly identified excitatory responses to a panel of carboxylic acids in a neuron that was tentatively identified as a deterrent neuron [29] . Carboxylic acids have also been shown to inhibit responses of sweet- and salt-sensing taste neurons in larger flies [30] , [31] , [32] , suggesting that this class of chemicals may be sensed by its activity on multiple categories of taste neurons. Acid tastants are found in common food sources of the fly, including over-ripe or rotting fruit [33] , but whether or not the Drosophila gustatory system detects acids has not yet been investigated. Here, we identify the cellular basis of acid taste in Drosophila . Using a panel of fruit carboxylic acids, we find that flies reject acidic stimuli in a pH-dependent manner. Electrophysiological analysis reveals that this class of tastants is detected by a subset of bitter taste neurons. Moreover, in the context of mixtures with sucrose, we find that acid tastants are also sensed by sweet taste neurons via inhibition of their response to sugar. Flies in which bitter taste neurons are genetically silenced have reduced aversion to acid–sucrose mixtures, showing that bitter taste neurons are necessary for rejection of acids. However, consistent with our electrophysiological analysis, mixtures of sucrose and carboxylic acids are still aversive to bitter-silenced flies, suggesting that the presence of acid tastants can be evaluated in the absence of a canonical deterrent neuron. In addition, we find that sweet neuron inhibition by acid tastants can be overcome by an increase in sugar concentration. We posit that the two independent sweet and bitter neuron mechanisms for sensing acids act in concert to convey the palatability of acidic food sources. Flies reject carboxylic acids in taste behaviour assays To identify taste responses to acids, we examined behaviours to four carboxylic acids that are found in fruit and vinegar. We first tested whether acids could evoke proboscis extension, a sign of food acceptance, upon stimulation of taste sensilla on the surface of the fly labellum. Preliminary tests showed that carboxylic acids failed to evoke proboscis extension when tested alone, similar to what has been observed for other classes of noxious stimuli, including allelochemicals and alkaloids [34] . We therefore tested if the presence of acids could suppress acceptance of sucrose, which stimulates a robust proboscis extension by itself. All four of the tested carboxylic acids were capable of blocking proboscis extension to sucrose ( Fig. 1a ), suggesting that the gustatory system harbours the ability to sense acidic compounds. We confirmed taste aversion for these carboxylic acids using an independent feeding preference assay. In a series of binary choice experiments in which flies were tested for preference between 1 mM sucrose and mixtures of 5 mM sucrose with acids, we found that sucrose–acid mixtures were rejected as the concentration of acid was increased ( Fig. 1b ). Benedict’s qualitative tests confirmed that the decreased preference for sucrose–acid mixtures was not owing to the hydrolysis of sucrose into fructose and glucose. 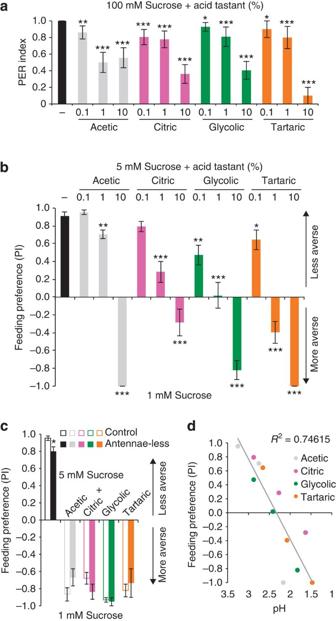Figure 1: Common fruit acids inhibitDrosophilataste behaviours. (a) Proboscis extension responses of wild-type flies to 100 mM sucrose alone (–) or in mixtures with indicated acids.n=32 (–),n=18 (acetic),n=18 (citric),n=21 (glycolic) andn=10 (tartaric). *P<0.05, **P<0.01, ***P<0.001, versus 100 mM sucrose, Student’st-test. For each stimulus, independent trials were conducted over 2–6 days. (b) Results of binary choice assays using indicated mixed stimuli tested against 1 mM sucrose.n=10 (sucrose control),n=6–10 (acetic),n=16–17 (citric),n=7 (glycolic) andn=7 (tartaric). *P<0.05, **P<0.01, ***P<0.001, versus 5 mM sucrose, Student’st-test. For each acid tastant series, independent trials were performed on 2–5 days. (c) Feeding preference of wild-type flies with antennae (control) and those with antennae removed surgically (antennae-less). Named acids were tested at 10%. For control, antennae-less:n=8, 9 (sucrose);n=6, 6 (acetic);n=6, 7 (citric);n=6, 6 (glycolic); andn=8, 6 (tartaric). The asterisk indicates significant difference in feeding preference versus control,P=0.025, Student’st-test. For each stimulus, independent trials were performed over 1–3 days. (d). Scatter plot of behavioural data inbagainst pH of the stimulus mixtures. Two pH measurements were taken and averaged for each stimulus solution. Linear best fit andR2value were calculated in Excel. Error bars, s.e.m. Figure 1: Common fruit acids inhibit Drosophila taste behaviours. ( a ) Proboscis extension responses of wild-type flies to 100 mM sucrose alone (–) or in mixtures with indicated acids. n =32 (–), n =18 (acetic), n =18 (citric), n =21 (glycolic) and n =10 (tartaric). * P <0.05, ** P <0.01, *** P <0.001, versus 100 mM sucrose, Student’s t -test. For each stimulus, independent trials were conducted over 2–6 days. ( b ) Results of binary choice assays using indicated mixed stimuli tested against 1 mM sucrose. n =10 (sucrose control), n =6–10 (acetic), n =16–17 (citric), n =7 (glycolic) and n =7 (tartaric). * P <0.05, ** P <0.01, *** P <0.001, versus 5 mM sucrose, Student’s t -test. For each acid tastant series, independent trials were performed on 2–5 days. ( c ) Feeding preference of wild-type flies with antennae (control) and those with antennae removed surgically (antennae-less). Named acids were tested at 10%. For control, antennae-less: n =8, 9 (sucrose); n =6, 6 (acetic); n =6, 7 (citric); n =6, 6 (glycolic); and n =8, 6 (tartaric). The asterisk indicates significant difference in feeding preference versus control, P =0.025, Student’s t -test. For each stimulus, independent trials were performed over 1–3 days. ( d ). Scatter plot of behavioural data in b against pH of the stimulus mixtures. Two pH measurements were taken and averaged for each stimulus solution. Linear best fit and R 2 value were calculated in Excel. Error bars, s.e.m. Full size image Many acids have pungent odours and a recent study identified acid-sensing olfactory neurons in the Drosophila antenna [35] . We therefore tested surgically antennectomized flies in feeding choice assays to determine the extent to which feeding aversion is dependent on acidic volatiles. Antennae-less flies showed a strong preference for 5 mM sucrose in the absence of acid (preference index for 5 mM sucrose=0.8±0.05, n =9 as compared with control flies with antennae 0.95±0.03, n =8; Fig. 1c ). Moreover, antennae-less flies avoided ingesting acid-laced sucrose to the same degree observed for their control siblings ( Fig. 1c ). Mean participation rates were also similar for control (37–89%) and antennae-less (36–78%) flies. Although antennae-less flies retain olfactory function in the maxillary palps, responses to acidic volatiles appear to be largely mediated by olfactory neurons in the antenna [35] . Thus, feeding aversion to carboxylic acids appears to be largely independent of olfactory input. Interestingly, feeding preference strongly correlated with pH of the tastant mixtures ( Fig. 1d ), raising the possibility that the fly gustatory system may sense free proton concentration, as has been observed for mammalian sour taste cells [28] . Carboxylic acids activate bitter taste neurons We next sought to identify the taste neurons responsible for acid recognition. Although taste neurons are located in a number of external and internal taste organs, we focused on the labellum, which is the best-characterized taste organ with respect to identification of individual taste hairs [36] , and their molecular and functional properties [4] , [37] . Each taste hair in the labellum can contain up to four gustatory neurons, of which one is tuned to sweet compounds and a second to bitter compounds [4] , [5] , [38] . Previous studies have shown that activation of bitter neurons drives behavioural taste aversion [3] , [39] , [40] . Given that acids are rejected in feeding choice assays, we tested the possibility that they directly activate bitter neurons. We surveyed responses of previously defined bitter sensilla of the labellum [4] to each of the four acids, which were tested at three different concentrations: 0.1, 1 and 10%. We also tested 10 mM caffeine (S-a, S-b, and I-b classes) or lobeline (I-a class) as positive controls for bitter neuron activation. We observed robust, concentration-dependent responses to carboxylic acids in S-b and I-b sensilla, which represent two of the four classes of labellar sensilla that house bitter-sensing taste neurons [4] . Our recordings revealed a neuron that fired in response to acids with a spike amplitude comparable to that seen in response to caffeine ( Fig. 2a ). Importantly, acid application did not significantly affect subsequent responsiveness to caffeine, indicating that acidic tastants were not damaging taste neurons in the sensillum ( Fig. 2b ). Stronger responses were elicited in the S-b class as compared with the I-b class, but in both cases the responses increased with higher acid concentrations ( Fig. 2c ). Consistent with the results of the feeding choice experiments, the neuronal firing rates in S-b and I-b sensilla were inversely correlated with pH of carboxylic acid tastants ( Fig. 2d ). Responses were also observed from the other bitter sensilla, S-a and I-a, but they were generally weaker and did not exhibit consistent concentration dependence ( Fig. 2e ) or strong correlation with acidic pH ( Fig. 2f ), suggesting that they have little if any role in acid detection. 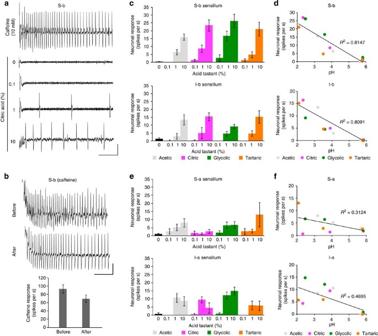Figure 2: Fruit acid tastants activate a subset of bitter neurons. (a) Representative traces of recordings obtained from S-b labellar sensilla of wild-type flies. Vertical bar, 1 mV; horizontal bar, 100 ms. (b) Representative 10 mM caffeine traces and mean firing rates of the bitter neuron obtained before and after stimulation with acid tastants.n=9.P=0.305, Student’st-test. Independent recordings were acquired over 2 days. Vertical bar, 1 mV; horizontal bar, 100 ms. (c) Mean responses of S-b and I-b classes of bitter-responsive sensilla to indicated acid tastants and 30 mM tricholine citrate electrolyte control (0). S-b:n=30 (‘0’ control),n=9–14 (acetic),n=10–11 (citric),n=8–9 (glycolic) andn=10–11 (tartaric). I-b:n=22 (‘0’ control),n=6–12 (acetic),n=6–10 (citric),n=7–10 (glycolic) andn=9–10 (tartaric). For each sensillum-stimulus series, independent recordings were acquired over 2–6 days. (d) Scatter plots of mean responses of S-b and I-b sensilla to acid tastants tested at 0.1%, 1% and 10% fromc, against pH of the stimulus mixtures. Three independent pH measurements were taken and averaged for each stimulus solution. Best fit lines andR2values were calculated in Excel. (e) Mean responses of wild-type S-a and I-a classes of bitter-responsive sensilla to indicated acid tastants and 30 mM tricholine citrate electrolyte alone (control). S-a:n=29 (‘0’ control),n=8–14 (acetic),n=10–14 (citric),n=8–11 (glycolic) andn=9–11 (tartaric); I-a:n=7 (‘0’ control),n=9–10 (acetic),n=8–9 (citric),n=9 (glycolic) andn=9 (tartaric). For each sensillum-stimulus series, independent recordings were acquired over 2–6 days. (f) Scatter plots of mean responses of indicated sensilla to acid tastants tested at 0.1, 1 and 10% against pH of the stimulus mixtures. Three independent pH measurements were taken and averaged for each stimulus solution. Best fit lines andR2values were calculated in Excel. Error bars, s.e.m. Figure 2: Fruit acid tastants activate a subset of bitter neurons. ( a ) Representative traces of recordings obtained from S-b labellar sensilla of wild-type flies. Vertical bar, 1 mV; horizontal bar, 100 ms. ( b ) Representative 10 mM caffeine traces and mean firing rates of the bitter neuron obtained before and after stimulation with acid tastants. n =9. P =0.305, Student’s t -test. Independent recordings were acquired over 2 days. Vertical bar, 1 mV; horizontal bar, 100 ms. ( c ) Mean responses of S-b and I-b classes of bitter-responsive sensilla to indicated acid tastants and 30 mM tricholine citrate electrolyte control (0). S-b: n =30 (‘0’ control), n =9–14 (acetic), n =10–11 (citric), n =8–9 (glycolic) and n =10–11 (tartaric). I-b: n =22 (‘0’ control), n =6–12 (acetic), n =6–10 (citric), n =7–10 (glycolic) and n =9–10 (tartaric). For each sensillum-stimulus series, independent recordings were acquired over 2–6 days. ( d ) Scatter plots of mean responses of S-b and I-b sensilla to acid tastants tested at 0.1%, 1% and 10% from c , against pH of the stimulus mixtures. Three independent pH measurements were taken and averaged for each stimulus solution. Best fit lines and R 2 values were calculated in Excel. ( e ) Mean responses of wild-type S-a and I-a classes of bitter-responsive sensilla to indicated acid tastants and 30 mM tricholine citrate electrolyte alone (control). S-a: n =29 (‘0’ control), n =8–14 (acetic), n =10–14 (citric), n =8–11 (glycolic) and n =9–11 (tartaric); I-a: n =7 (‘0’ control), n =9–10 (acetic), n =8–9 (citric), n =9 (glycolic) and n =9 (tartaric). For each sensillum-stimulus series, independent recordings were acquired over 2–6 days. ( f ) Scatter plots of mean responses of indicated sensilla to acid tastants tested at 0.1, 1 and 10% against pH of the stimulus mixtures. Three independent pH measurements were taken and averaged for each stimulus solution. Best fit lines and R 2 values were calculated in Excel. Error bars, s.e.m. Full size image Subsets of bitter neurons are pH sensors Given the relationship of taste neuron responses to pH of carboxylic acids, we wanted to determine whether S-b and I-b sensilla could sense low pH. We therefore performed recordings using standardized hydrochloric acid (HCl) solutions at pH 2–6, as well as control 30 mM tricholine citrate electrolyte alone, which read at about pH 6.65 ( Fig. 3 ). We also tested the responses of S-a and I-a sensilla, which did not show strong responses to carboxylic acids, as well as L-type sensilla that lack canonical bitter neurons [4] to verify lack of pH activation in them. Overall, our results revealed defined subpopulations of bitter taste neurons that detect acidic pH. 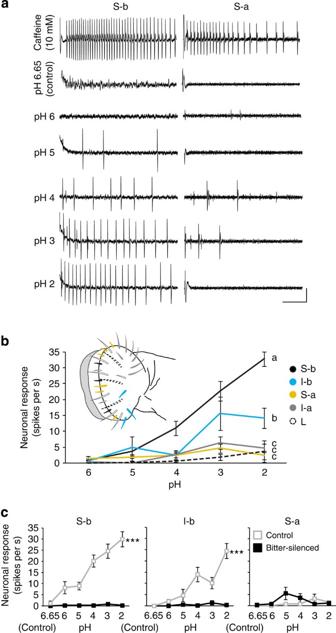Figure 3: Bitter taste neurons are activated by acidic pH. (a) Representative traces of HCl responses obtained from S-b and S-a sensilla of wild-type flies. Vertical bar, 1 mV; horizontal bar, 100 ms. (b) Mean responses of five classes of labellar sensilla to solutions of HCl at indicated pH; corresponding sensillar classes are indicated in the schematic of the labellum.n=12 (S-b),n=9 (I-b),n=9 (S-a),n=5–10 (I-a) andn=10 (L). Lines with different letters are significantly different,P<0.001 (S-b),P<0.001 (I-b),P=0.861 (S-a),P=0.478 (I-a) versus L-type, two-way ANOVA with Tukey’spost hocanalysis. For each sensillum, independent recordings were acquired over 2–3 days. (c) Mean responses to 30 mM tricholine citrate electrolyte alone (pH 6.65, control) and standardized HCl solutions in electrolyte (pH 2–6) of indicated sensilla in control (Gr89a-GAL4/+;+/TM3) and bitter-silenced (Gr89a-GAL4/+;UAS-Kir2.1/TM3) flies. Control:n=12 (S-b),n=9 (I-b) andn=5 (S-a); bitter-silenced:n=10 (S-b),n=10 (I-b) andn=5 (S-a). ***P<0.001, two-way ANOVA with pairwise comparisons. For each sensillum, independent recordings were acquired over 3–5 days. Figure 3: Bitter taste neurons are activated by acidic pH. ( a ) Representative traces of HCl responses obtained from S-b and S-a sensilla of wild-type flies. Vertical bar, 1 mV; horizontal bar, 100 ms. ( b ) Mean responses of five classes of labellar sensilla to solutions of HCl at indicated pH; corresponding sensillar classes are indicated in the schematic of the labellum. n =12 (S-b), n =9 (I-b), n =9 (S-a), n =5–10 (I-a) and n =10 (L). Lines with different letters are significantly different, P <0.001 (S-b), P <0.001 (I-b), P =0.861 (S-a), P =0.478 (I-a) versus L-type, two-way ANOVA with Tukey’s post hoc analysis. For each sensillum, independent recordings were acquired over 2–3 days. ( c ) Mean responses to 30 mM tricholine citrate electrolyte alone (pH 6.65, control) and standardized HCl solutions in electrolyte (pH 2–6) of indicated sensilla in control ( Gr89a-GAL4 /+;+/ TM3 ) and bitter-silenced ( Gr89a-GAL4 /+; UAS-Kir2.1 / TM3 ) flies. Control: n =12 (S-b), n =9 (I-b) and n =5 (S-a); bitter-silenced: n =10 (S-b), n =10 (I-b) and n =5 (S-a). *** P <0.001, two-way ANOVA with pairwise comparisons. For each sensillum, independent recordings were acquired over 3–5 days. Full size image First, our recordings confirmed that neurons in S-b and I-b sensilla were activated by acidic pH ( Fig. 3a ). Second, our analysis showed that S-a and I-a sensilla were unresponsive to acidic pH, corroborating heterogeneity in pH sensitivity across sensillar classes ( Fig. 3a ), as has been observed for bitter compounds [4] . Third, we found that acidic pH solutions were not able to activate neurons in L-type sensilla ( Fig. 3b ), supporting the involvement of bitter taste neurons that are absent in these sensilla. Indeed, genetic silencing of all labellar bitter taste neurons by expressing an inwardly rectifying potassium channel, Kir2.1, under the control of Gr89a-GAL4 [4] resulted in loss of pH responses in S-b and I-b sensilla ( P <0.001; Fig. 3c ), but had no effect on the weak pH response in S-a ( P =0.126; Fig. 3c ). Thus, acid taste appears to be encoded by a subset of bitter neurons in the periphery. To begin to investigate the molecular mechanism of pH detection in bitter taste neurons, we examined pH responses of S-b sensilla in mutant flies lacking candidate receptor genes. We tested Ir64a mutants, which lack an ionotropic receptor necessary for acid sensing in olfactory neurons [35] , and found no reduction in the sensitivity of their taste neurons to low pH ( Fig. 4a ); in fact, there was a small but significant increase in the level of acidic pH response, which may be attributable to differences in the genetic background. No significant differences in low pH responses were observed also for mutants lacking Gr33a, a receptor that is broadly required for responses to various noxious tastants [11] , and painless, a cation channel involved in aversion to wasabi [14] . Another likely candidate pH receptor was TrpA1 [41] , which is expressed in bitter taste neurons in Drosophila [15] , [16] . However, pH responses of TrpA1 mutants were also not significantly different from those of wild-type controls ( Fig. 4a ). Recordings from flies lacking a PKD-like gene Pkd2 , related to PKD1L3 and PKD2L1 [25] , [26] channels that are expressed in mammalian sour taste cells, showed that it is not necessary for pH-dependent activity in S-b sensilla ( Fig. 4a ). 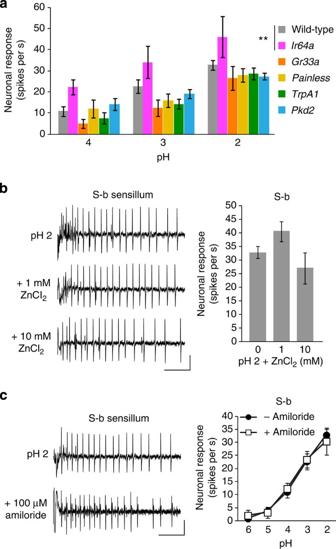Figure 4: Candidate receptor mutants or inhibitors do not reduce acid response. (a) Mean pH responses of S-b sensilla in genotypes as indicated. Genotypes were:w1118(wild-type)n=12,Ir64aMB05283(Ir64a)n=5,Gr33a1(Gr33a)n=6,painEP2621(painless)n=6,TrpA11(TrpA1)n=6 andPkd21(Pkd2)n=7. **P<0.01 versus wild-type, two-way ANOVA with Tukey’spost hocanalysis. For each genotype, at least two independent flies were tested on the same day. Error bars, s.e.m. (b,c) Representative traces and mean responses of wild-type S-b labellar sensilla to standardized HCl solutions at indicated pH alonen=12 (0 or −) or in mixtures with ZnCl2(n=10 for 1 mM ZnCl2andn=4 for 10 mM ZnCl2) or amiloride hydrochloriden=5–7. Neither ZnCl2(Student’st-test) nor amiloride hydrochloride (two-way ANOVA with pairwise comparisons) caused any change in pH response. Vertical bar, 1 mV; horizontal bar, 100 ms. Error bars, s.e.m. Figure 4: Candidate receptor mutants or inhibitors do not reduce acid response. ( a ) Mean pH responses of S-b sensilla in genotypes as indicated. Genotypes were: w 1118 (wild-type) n =12, Ir64a MB05283 ( Ir64a ) n =5, Gr33a 1 ( Gr33a ) n =6, pain EP2621 ( painless ) n =6, TrpA1 1 ( TrpA1 ) n =6 and Pkd2 1 ( Pkd2 ) n =7. ** P <0.01 versus wild-type, two-way ANOVA with Tukey’s post hoc analysis. For each genotype, at least two independent flies were tested on the same day. Error bars, s.e.m. ( b , c ) Representative traces and mean responses of wild-type S-b labellar sensilla to standardized HCl solutions at indicated pH alone n =12 (0 or −) or in mixtures with ZnCl 2 ( n =10 for 1 mM ZnCl 2 and n =4 for 10 mM ZnCl 2 ) or amiloride hydrochloride n =5–7. Neither ZnCl 2 (Student’s t -test) nor amiloride hydrochloride (two-way ANOVA with pairwise comparisons) caused any change in pH response. Vertical bar, 1 mV; horizontal bar, 100 ms. Error bars, s.e.m. Full size image A recent study showed that acid response in mammalian sour taste cells is inhibited by zinc chloride but not by amiloride hydrochloride [28] . However, we found that pH-evoked response in Drosophila S-b sensilla was refractory to both zinc ion ( P =0.074 for 1 mM, P =0.267 for 10 mM, Student’s t -test, Fig. 4b ) and amiloride ( P =0.948, analysis of variance (ANOVA), Fig. 4c ). Together with our mutant analyses, these results suggest that acidic pH is detected by a novel receptor that is expressed in a subset of bitter taste neurons. Acids inhibit sugar response of sweet neurons In natural food sources, Drosophila are likely to encounter carboxylic acids in the context of mixtures with compounds such as sugars. Previous studies have shown that chemosensory neuron responsiveness can be altered by the chemical context in which its stimulus is received [42] . In fact, carboxylic acids have been shown to inhibit the activity of salt taste neurons in the blowfly [29] , and pH effects have been characterized on sweet- and salt-sensing neurons in blowflies or fleshflies [30] , [31] , [43] . We therefore examined if sweet taste neuron response in Drosophila is affected by the presence of acid tastants. We performed recordings from L-type sensilla, which did not respond to acid tastants alone ( Fig. 3b and Fig. 5a ). For each sensillum, we first recorded the response to 100 mM sucrose and subsequently tested mixtures of sucrose with increasing concentrations of acids. Typically, a single acid–sucrose series was tested on each sensillum and recordings were concluded with a final application of 100 mM sucrose. There was a significant reduction in sucrose recovery after application of glycolic and tartaric acids, but the observed activity verified that the sucrose–acid mixtures did not result in severe neuronal injury or death ( Fig. 5b ). We found that sucrose response was inhibited by acid tastants in a concentration-dependent manner ( Fig. 5c ). The temporal dynamics of sweet neuron response, showing a high initial firing rate followed by a sustained lower rate of firing after a quick decay, revealed some variation in the effects of different acid tastants over time although the general patterns of inhibition were similar ( Fig. 5d ). 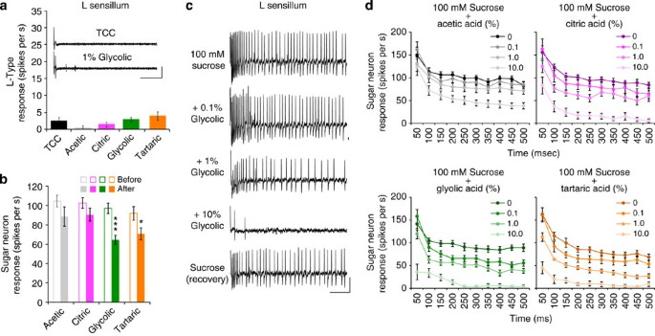Figure 5: Fruit acid tastants inhibit sucrose response of sweet taste neurons. (a) Mean responses of L-type sensilla to indicated acids at 1% in mixtures with 30 mM tricholine citrate electrolyte, which was also tested alone as control. Inset shows representative traces of recordings obtained from an L-type sensillum of a wild-type fly with electrolyte alone (control) or 1% glycolic acid. Vertical bar, 1 mV; horizontal bar, 100 ms.n=7 for all stimuli. Two independent flies were tested on the same day. (b) Mean sucrose response before and after acid–mixture recordings. In order of before, after:n=18,13 (acetic);n=20,19 (citric);n=13,13 (glycolic); andn=21,21 (tartaric). *P<0.05, ***P<0.001, Student’st-test. For each stimulus series, recordings were acquired over 4–10 days. (c) Representative traces of recordings from a single L-type sensillum of a wild-type fly with indicated stimuli. ‘Recovery’ shows response to 100 mM sucrose after testing the mixture with the highest concentration of glycolic acid. Vertical bar, 1 mV; horizontal bar, 100 ms. (d) Temporal dynamics of sweet neuron response in L-type sensilla to 100 mM sucrose alone or in mixtures with indicated concentrations of acid tastants. Action potentials were counted in 50-ms bins for the 500-ms period upon stimulus contact with the sensillum.n=10–13 (acetic),n=12–14 (citric),n=10–14 (glycolic) andn=11–15 (tartatic). For each stimulus series, recordings were acquired over 3–7 days. Figure 5: Fruit acid tastants inhibit sucrose response of sweet taste neurons. ( a ) Mean responses of L-type sensilla to indicated acids at 1% in mixtures with 30 mM tricholine citrate electrolyte, which was also tested alone as control. Inset shows representative traces of recordings obtained from an L-type sensillum of a wild-type fly with electrolyte alone (control) or 1% glycolic acid. Vertical bar, 1 mV; horizontal bar, 100 ms. n =7 for all stimuli. Two independent flies were tested on the same day. ( b ) Mean sucrose response before and after acid–mixture recordings. In order of before, after: n =18,13 (acetic); n =20,19 (citric); n =13,13 (glycolic); and n =21,21 (tartaric). * P <0.05, *** P <0.001, Student’s t -test. For each stimulus series, recordings were acquired over 4–10 days. ( c ) Representative traces of recordings from a single L-type sensillum of a wild-type fly with indicated stimuli. ‘Recovery’ shows response to 100 mM sucrose after testing the mixture with the highest concentration of glycolic acid. Vertical bar, 1 mV; horizontal bar, 100 ms. ( d ) Temporal dynamics of sweet neuron response in L-type sensilla to 100 mM sucrose alone or in mixtures with indicated concentrations of acid tastants. Action potentials were counted in 50-ms bins for the 500-ms period upon stimulus contact with the sensillum. n =10–13 (acetic), n =12–14 (citric), n =10–14 (glycolic) and n =11–15 (tartatic). For each stimulus series, recordings were acquired over 3–7 days. Full size image We next compared acid tastant-mediated inhibition of sweet taste neurons of L-, I- or S-type sensilla, which exhibit some quantitative variation in their responses to sugars [37] , and found little difference in the extent to which sucrose responses across these sensilla were reduced by the presence of citric or tartaric acid tastants ( Fig. 6a ). The occurrence of acid-mediated sweet neuron inhibition in sensilla that lack bitter neurons (L-type) suggested that it is independent of bitter neuron activation. To determine whether this is indeed the case, we examined sucrose response inhibition by citric and tartaric acids in I-type sensilla of bitter-silenced flies, in which the sweet neuron remains the sole functional neuron in the sensillum [4] , [44] . We measured responses to acid–sucrose mixtures and normalized each to baseline sucrose response obtained immediately before application of the mixed stimulus. A comparison of normalized responses across the two genotypes showed that acid-dependent inhibition was not significantly different in bitter-silenced flies as compared with sibling controls ( Fig. 6b ). These results substantiate an independent role for sweet taste neurons in assessing the value of acidic food sources. 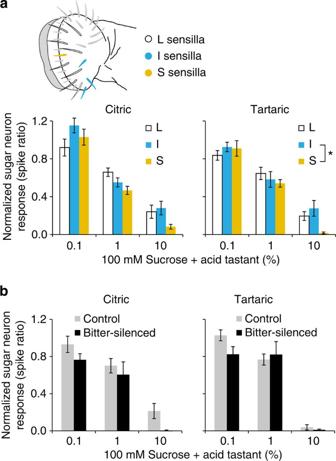Figure 6: Acid inhibition of sweet neurons is independent of bitter neurons. (a) Response of sweet taste neurons to sucrose–acid mixtures normalized to sucrose response. Baseline sucrose recordings were taken immediately before every application of a mixed stimulus. L-, I- and S-type sensilla that were chosen for recordings are indicated in the schematic on top. Citric:n=12–14 (L),n=10–11 (I) andn=9 (S); tartaric:n=11–15 (L),n=8–10 (I) andn=10 (S). *P=0.033, two-way ANOVA with Tukey’spost hocanalysis. (b) Normalized responses of sweet taste neurons in control (Gr89a-GAL4/+;+/GFP) and bitter-silenced (Gr89a-GAL4/+;UAS-Kir2.1/GFP) flies. Recordings were obtained from I-b sensilla. Citric:n=4–11 (control) andn=11–12 (bitter-silenced); tartaric:n=9–12 (control) andn=10–14 (bitter-silenced).P=0.853 (citric),P=0.294 (tartaric), two-way ANOVA with pairwise comparisons. For each genotype-stimulus series, recordings were acquired over 1–2 days. Error bars, s.e.m. Figure 6: Acid inhibition of sweet neurons is independent of bitter neurons. ( a ) Response of sweet taste neurons to sucrose–acid mixtures normalized to sucrose response. Baseline sucrose recordings were taken immediately before every application of a mixed stimulus. L-, I- and S-type sensilla that were chosen for recordings are indicated in the schematic on top. Citric: n =12–14 (L), n =10–11 (I) and n =9 (S); tartaric: n =11–15 (L), n =8–10 (I) and n =10 (S). * P =0.033, two-way ANOVA with Tukey’s post hoc analysis. ( b ) Normalized responses of sweet taste neurons in control ( Gr89a-GAL4 /+;+/ GFP ) and bitter-silenced ( Gr89a-GAL4 /+; UAS-Kir2.1 / GFP ) flies. Recordings were obtained from I-b sensilla. Citric: n =4–11 (control) and n =11–12 (bitter-silenced); tartaric: n =9–12 (control) and n =10–14 (bitter-silenced). P =0.853 (citric), P =0.294 (tartaric), two-way ANOVA with pairwise comparisons. For each genotype-stimulus series, recordings were acquired over 1–2 days. Error bars, s.e.m. Full size image Acids are rejected in the absence of functional bitter neurons We next asked whether inhibition of sweet neurons by acid tastants is behaviourally relevant. We measured behavioural responses in flies with genetically silenced bitter taste neurons in which UAS-Kir2.1 expression was driven by Gr89a-GAL4 , which is broadly expressed in all bitter neurons of the labellum [4] . Proboscis extension trials with sucrose–caffeine mixtures verified that caffeine aversion was impaired in bitter-silenced flies ( Fig. 7a ). However, these flies continued to reject sucrose–acid mixtures to the same extent observed for controls, with the exception of tartaric acid at the highest concentration tested ( Fig. 7a ). In agreement with the results of proboscis extension tests, bitter-silenced flies retained the ability to avoid feeding on sucrose–acid mixtures, although the reduced sensitivity of these flies as compared with control siblings supports a partial but significant role for bitter neurons in driving acid deterrence behaviour ( Fig. 7b ). Consistent with our analysis of carboxylic acid-dependent inhibition of sweet neurons, feeding avoidance was linked to acid tastant concentration even in the absence of functional bitter neurons, and was largely independent of antennal olfactory input ( Fig. 7b ). The results of the two independent assays support the view that taste-driven behaviours to carboxylic acids are driven by their action on both sweet and bitter neurons. 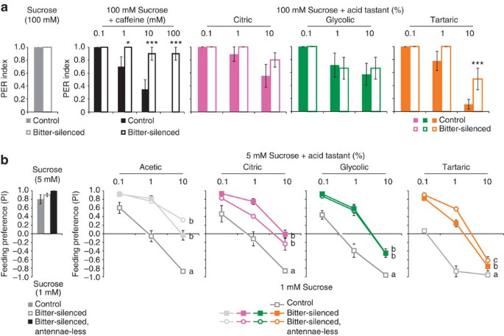Figure 7: Bitter-silenced flies retain the ability to reject acidic sugar stimuli. (a) Proboscis extension responses of control (Gr89a-GAL4/+;+/GFP) and bitter-silenced (Gr89a-GAL4/+;UAS-Kir2.1/GFP) flies to 100 mM sucrose alone or in mixtures with caffeine or acid tastants. Sucrose:n=44 (control) andn=46 (bitter-silenced); caffeine:n=10 (control) andn=10 (bitter-silenced); citric:n=9 (control) andn=10 (bitter-silenced); glycolic:n=7 (control) andn=9 (bitter-silenced); tartaric:n=9 (control) andn=9 (bitter-silenced). *P<0.05, ***P<0.005, bitter-silenced versus control, two-way ANOVA with pairwise comparisons. For each genotype-stimulus combination, independent trials were performed on 2 days. (b) Feeding preferences of control (Gr89a-GAL4/+;+/TM3), bitter-silenced (Gr89a-GAL4/+;UAS-Kir2.1/TM3), and bitter-silenced, antennae-less (Gr89a-GAL4/+;UAS-Kir2.1/TM3with antennae removed surgically) flies. Stimulus and assay conditions were as inFig. 1b, except that flies were starved for 15 hours prior to testing. In the order of control, bitter-silenced and bitter-silenced, antennae-less:n=11, 13, 3 (sucrose control);n=7–8, 7–8, 3 (acetic);n=7, 7–8, 3 (citric);n=7, 7, 3 (glycolic),n=8–10, 8–10, 3 (tartaric). Lines with different letters are significantly different,P<0.001 for all comparisons, exceptP=0.031 for b versus c lines for tartaric acid, two-way ANOVA with Tukey’spost hocanalysis. For each genotype-stimulus combination, independent trials were performed on 2 days. Error bars, s.e.m. Figure 7: Bitter-silenced flies retain the ability to reject acidic sugar stimuli. ( a ) Proboscis extension responses of control ( Gr89a-GAL4 /+;+/ GFP ) and bitter-silenced ( Gr89a-GAL4 /+; UAS-Kir2.1 / GFP ) flies to 100 mM sucrose alone or in mixtures with caffeine or acid tastants. Sucrose: n =44 (control) and n =46 (bitter-silenced); caffeine: n =10 (control) and n =10 (bitter-silenced); citric: n =9 (control) and n =10 (bitter-silenced); glycolic: n =7 (control) and n =9 (bitter-silenced); tartaric: n =9 (control) and n =9 (bitter-silenced). * P <0.05, *** P <0.005, bitter-silenced versus control, two-way ANOVA with pairwise comparisons. For each genotype-stimulus combination, independent trials were performed on 2 days. ( b ) Feeding preferences of control ( Gr89a-GAL4 /+;+/ TM3 ), bitter-silenced ( Gr89a-GAL4 /+; UAS-Kir2.1 / TM3 ), and bitter-silenced, antennae-less ( Gr89a-GAL4 /+; UAS-Kir2.1 / TM3 with antennae removed surgically) flies. Stimulus and assay conditions were as in Fig. 1b , except that flies were starved for 15 hours prior to testing. In the order of control, bitter-silenced and bitter-silenced, antennae-less: n =11, 13, 3 (sucrose control); n =7–8, 7–8, 3 (acetic); n =7, 7–8, 3 (citric); n =7, 7, 3 (glycolic), n =8–10, 8–10, 3 (tartaric). Lines with different letters are significantly different, P <0.001 for all comparisons, except P =0.031 for b versus c lines for tartaric acid, two-way ANOVA with Tukey’s post hoc analysis. For each genotype-stimulus combination, independent trials were performed on 2 days. Error bars, s.e.m. Full size image Sweet neuron activity relies on both sugar content and acidity Our observation that both bitter neuron activation and sweet neuron inhibition coordinate to allow the fly to reject carboxylic acids raised questions about how Drosophila are driven to consume ripe or over-ripe fruits that can have an acid content comparable to that of unripe fruit [33] . To investigate this, we wanted to determine whether an increase in sugar concentration, generally associated with ripening, could overcome acid-evoked inhibition in sweet neurons. We obtained recordings from sweet neurons in L-type sensilla using mixtures of 10% citric acid with sucrose ( Fig. 8a ), and found that there was an increase in the firing rate of the sweet neuron with increasing concentrations of sucrose in the sucrose–acid mixtures ( Fig. 8b ). For each stimulus mixture, we normalized the response to that of sucrose at the same concentration, which was obtained immediately before the acid–sucrose recording. A comparison of the normalized responses showed that the strength of acid-evoked inhibition was weaker with higher sugar content in the mixed stimuli ( Fig. 8b ). 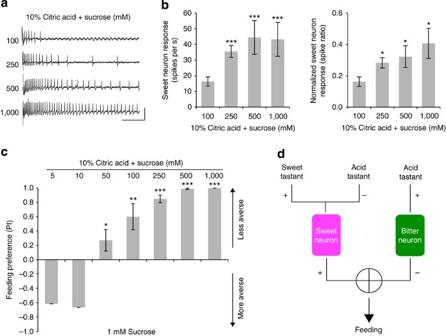Figure 8: Acid inhibition of sweet neurons is relieved by increases in sucrose concentration. (a) Representative traces of recordings from a single L-type sensillum of a wild-type fly. Vertical bar, 1 mV; horizontal bar, 100 ms. (b) Mean responses (left) and responses normalized to the corresponding concentration of sucrose (right) obtained for sweet taste neurons in L-type sensilla.n=10–15. *P<0.05, ***P<0.005, versus mixture with 100 mM sucrose, Student’st-test. Independent recordings were acquired over 2 days. (c) Results of binary choice assays using indicated mixed stimuli tested against 1 mM sucrose.n=3–10. *P<0.05, **P<0.01, ***P<0.005, Student’st-test. Error bars, s.e.m. Independent trials were performed over 2 days. (d) A model for the detection of acid tastants by theDrosophilataste system. Figure 8: Acid inhibition of sweet neurons is relieved by increases in sucrose concentration. ( a ) Representative traces of recordings from a single L-type sensillum of a wild-type fly. Vertical bar, 1 mV; horizontal bar, 100 ms. ( b ) Mean responses (left) and responses normalized to the corresponding concentration of sucrose (right) obtained for sweet taste neurons in L-type sensilla. n =10–15. * P <0.05, *** P <0.005, versus mixture with 100 mM sucrose, Student’s t -test. Independent recordings were acquired over 2 days. ( c ) Results of binary choice assays using indicated mixed stimuli tested against 1 mM sucrose. n =3–10. * P <0.05, ** P <0.01, *** P <0.005, Student’s t -test. Error bars, s.e.m. Independent trials were performed over 2 days. ( d ) A model for the detection of acid tastants by the Drosophila taste system. Full size image We next wanted to test whether flies would choose to consume low pH foods if the sugar content were higher. We performed a series of feeding choice experiments in which flies were tested for preference between 1 mM sucrose and 10% citric acid with varying concentrations of sucrose. As before, we found that flies rejected a mixture of 10% citric acid and 5 mM sucrose ( Fig. 8c ). However, increasing the amount of sucrose caused a shift in behaviour, and flies displayed a positive behavioural valence for mixtures with sucrose at a concentration ≥50 mM ( Fig. 8c ). Taken together, our results suggest that sweet taste neuron activity can convey the palatability of food sources by integrating information about sugar and carboxylic acid content. Our study demonstrates two independent cellular mechanisms by which a previously uncharacterized class of taste stimuli are detected and evaluated by the Drosophila gustatory system ( Fig. 8d ). We propose that the action of carboxylic acid tastants on both sweet-sensing acceptance neurons and bitter-sensing deterrent neurons allows the animal to assess and modulate the risk of ingesting acidic food sources. Sour taste is described as one of the five basic taste modalities and acid sensing is therefore an important feature of the taste system. The Drosophila taste system is functionally organized in a manner that displays remarkable parallels to that of mammals, with separate cellular sensors for sweet, bitter and salt taste categories [1] . Here, we find that although flies do not appear to have a dedicated population of ‘sour’ taste cells, acidity evokes excitatory responses in a defined subset of bitter taste cells. Thus, there is an anatomical basis for discrimination of acid taste from that of sweet, salt and water taste in the fly. It will be interesting to determine whether the fly can separate acid and bitter tastes as well. Sour taste receptors have not been characterized in any organism. Although sour taste receptor cells are specifically labelled by PKD2L1 and PKD1L3 [25] , [26] , heterologous expression of the two channels suggests that this complex is activated upon removal of acid tastants [45] , and is not necessary for acid-evoked excitation in sour taste cells [27] . Another member of the TRP family, TrpA1, is expressed in acid-responsive trigeminal nociceptive neurons. In this instance, the relevant excitatory cue for TrpA1 appears to be intracellular acidification caused by weak acids such as acetic acid [41] . A more recent pharmacological analysis implicates the presence of a Zn 2+ -sensitive receptor that is activated by free protons in sour taste cells [28] , but a candidate receptor protein has not been found. Our results support the view that the fly taste receptor for acidic pH is not among those with previously identified roles in detecting noxious tastants, which include the Gr33a, TrpA1 and painless receptors. Moreover, the activity of the fly pH receptor is not blocked by amiloride, an inhibitor that broadly affects acid-sensing ion channels [46] , or Zn 2+ . Our finding that low pH response is specific to a subpopulation of bitter neurons offers the means to identify novel receptors that are restricted to those cells. Based on the widespread occurrence of acidic stimuli, it is no surprise that they have been identified as important chemical cues for many insects. Carboxylic acids are found in many fruits and food sources, and at least in one instance of a specialist, Drosophila sechellia , the fly has adapted to the presence of hexanoic and octanoic acids to exploit a narrow food and oviposition source [47] , [48] . Carboxylic acids are also thought to be important as human host-recognition cues for mosquitoes [49] , [50] , although the role of the gustatory system in detecting carboxylic acid components of human sweat has not yet been investigated. Our results raise the possibility that evolutionary variations in acid detection by insect taste systems may depend on altered activity in both bitter and sweet taste neurons. Recent studies expose an increasingly sophisticated role of sensory neuron function and communication in encoding the context of chemical stimuli. Such mechanisms break the neat compartmentalization of sensory cells at the periphery and have been found to act in both cell-autonomous and non-autonomous ways. For example, the response of the cell to one stimulus can be modified by the presence of other stimuli [42] . Also, an activated cell can influence the firing frequency of other cells in the same grouped unit by non-synaptic communication [51] . Here, we report that sweet neuron activity reflects the concentrations of both sugar and acid tastants, independent of acid-evoked excitation of bitter neurons. Such integration of information about different taste categories at the periphery may allow the fly to quickly calibrate the risk of ingesting nutritious foods that also contain potentially harmful substances without the involvement of central processing mechanisms. Whether the inhibition of sweet neurons by acid tastants occurs by direct action on sweet taste receptors or via more general mechanisms remains to be determined. It is possible that carboxylic acids also act on other classes of taste neurons such as the salt- or water-sensing neurons. Nonetheless, an independent role for an acceptance taste neuron in sensing acid tastants suggests a mechanism for facilitating meticulous evaluation of mixed stimuli within the constraints of a labelled-line coding system. The fly might use such mechanisms to better calculate the risk of consuming tainted food sources, which might otherwise be avoided irrespective of their nutritious value. Fly stocks Flies were raised on standard cornmeal–dextrose–agar diet at 25 °C. Wild-type flies were w 1118 . Mutant fly stocks were obtained from the Bloomington Stock Center: Ir64a [MB05283] (BL24610), Gr33a 1 (BL31427), TrpA1 1 (BL26504), and pain [EP2621] (BL28799), and Pkd2 1 (BL24495). UAS-Kir2.1 flies were kindly provided by K Scott (University of California, Berkeley). Solutions Tastants were obtained from Sigma Aldrich at the highest purity available. Organic acid-containing solutions were prepared on the day of use. Standardized pH solutions with HCl were stored for 1 week at room temperature. Behaviour For feeding preference assays, adult flies aged 3–7 days were sorted and housed in fresh food vials for 1–2 days; one vial was prepared for every trial and contained ten males and ten females. Flies were then starved for 24 h in vials with water-soaked Kimwipes. Feeding assay plates were prepared a few hours before the experiment and dotted with 9 spots of 10 μl of each stimulus solution in 0.75% agarose [9] . Tastants were mixed in with melted agarose and dispensed immediately. Flies were anesthetized momentarily with CO 2 , transferred to feeding plates and allowed to feed for 2 h in a dark, humidified chamber, after which they were frozen and scored within 48 h for the colour of their abdomens. For experiments with antennectomized flies, antennae were removed surgically and flies were allowed to recover for 48 h before they were starved and tested as above. Trials in which fewer than 25% flies had participated in feeding were discarded. Preference index was calculated as: Participation was calculated as: # indicates the number of flies with indicated abdomen colour. For proboscis extension response assays, 5–10-day-old male flies were starved as above. Individual flies were then trapped in cut 20-μl pipette tips such that their heads were exposed. Flies were first allowed to drink water to satiation; any flies that did not cease drinking were discarded and only those that subsequently responded to 100 mM sucrose were selected for further experimentation. Acid–sucrose mixtures were tested from lowest to highest acid concentration with water presented between stimuli. Scores were assigned as follows: 1=proboscis extension with drinking, 0.5=partial extension or extension with immediate retraction and 0=no extension. Hundred millimolar sucrose was also tested at the end of the acid series and only flies that responded were used for data analysis. Electrophysiology Single-sensillum recordings with acid tastants were performed using the tip-recording method [52] with 30 mM tricholine citrate as the electrolyte [53] . Recordings were obtained from male flies aged 3–10 days. In every case, a positive control of caffeine or lobeline, as appropriate, was tested before and after recordings with acid tastants. For recordings with standardized pH solutions, each sensillum was first tested with electrolyte alone as a control (pH 6.65), followed by HCl solutions of pH 2–6 in descending order. Neuronal responses were quantified by doubling the number of spikes in the 0–500 ms window upon contact with the stimulus. Recordings with sucrose–acid mixtures were obtained from male flies aged 3–10 days. Sensilla were first tested with 100 mM sucrose and only those that had initial responses ≥50 spikes per second (L-type) or ≥30 spikes per second (I- and S-type) were used. Response to 100 mM sucrose was tested before each stimulus in the acid–mixture series, which was presented from lowest to highest acid concentration. A sucrose recording was also taken at the end, and only those sensilla with responses within two s.d.’s of the mean initial response were used for data analysis. With the exception of results shown in Fig. 4d , neuronal responses were quantified by doubling the number of spikes in the 0–500 ms window upon contact with the stimulus. Statistical analysis Unless otherwise indicated, for behaviour experiments arcsine-transformed data were analysed using two-way ANOVA and Tukey’s post hoc analysis or pairwise comparisons. Electrophysiology data were analysed with two-way ANOVA followed by pairwise comparisons to determine significance at single concentrations, for all except pan-sensillar sucrose inhibition and pH activation for which Tukey’s post hoc tests were performed instead of pairwise comparisons. For all graphs, error bars indicate s.e.m. How to cite this article: Charlu, S. et al. Acid sensing by sweet and bitter taste neurons in Drosophila melanogaster . Nat. Commun. 4:2042 doi: 10.1038/ncomms3042 (2013).